Direct observation of half-metallicity in the Heusler compound Co2MnSi Ferromagnetic thin films of Heusler compounds are highly relevant for spintronic applications owing to their predicted half-metallicity, that is, 100% spin polarization at the Fermi energy. However, experimental evidence for this property is scarce. Here we investigate epitaxial thin films of the compound Co 2 MnSi in situ by ultraviolet-photoemission spectroscopy, taking advantage of a novel multi-channel spin filter. By this surface sensitive method, an exceptionally large spin polarization of ( ) % at room temperature is observed directly. As a more bulk sensitive method, additional ex situ spin-integrated high energy X-ray photoemission spectroscopy experiments are performed. All experimental results are compared with advanced band structure and photoemission calculations which include surface effects. Excellent agreement is obtained with calculations, which show a highly spin polarized bulk-like surface resonance ingrained in a half metallic bulk band structure. The magnitude of the room temperature spin polarization of ferromagnetic materials is a key property for their application in spin transport-based electronics [1] . Values close to 100% were observed for the metastable CrO 2 (ref. 2 ) and for Fe 3 O 4 (ref. 3 ), but these materials did not allow for large spin transport effects and are not compatible with applications. Thus intermetallic Heusler compounds [4] with their predicted half-metallic properties, that is, 100% spin polarization at the Fermi energy, moved into the focus of interest. In addition to being interesting for applications, intermetallic Heusler materials are a test for modern band structure calculations for materials with electronic correlations of moderate strength [5] . By means of various band structure methods many Heusler compounds have been predicted to be 100% spin polarized. For instance, for Co 2 MnSi, several publications predict half-metallicity, with different sizes of the minority charge carrier band gap and position of the Fermi energy [6] , [7] , [8] , [9] , [10] , [11] , [12] . These predictions have initiated major efforts to incorporate Heusler electrodes in magnetic tunnel junction devices, which are used for applications such as magnetic hard disc read heads and memory cells [1] . The magnetoresistance effect of planar tunnelling junctions between ferromagnetic electrodes is often related to the spin polarization by the application of the Jullière model [13] , which is justified only if the translational symmetry in the tunnelling process is completely broken. Employing AlO x tunnelling barriers it is generally assumed that this condition is fulfilled. However, typically the highest spin polarizations of Heusler compounds obtained by this method amount to 60–70% at low temperatures [14] , [15] , with a single exception of 83–89% at 2 K, which collapses to ≃ 50% at room temperature [16] . In junctions with epitaxial symmetry filtering MgO (ref. 17 ) and MgAl 2 O 4 (ref. 18 ) barriers, magnetoresistances comparable to junctions with conventional three-dimensional-metal ferromagnetic electrodes [19] were obtained. Thus up to now, especially at room temperature, Heusler compounds did not show to be superior to conventional ferromagnets such as CoFeB. Nevertheless, compared with the half-metallic oxides CrO 2 and Fe 3 O 4 much larger tunnelling magnetoresistances were obtained as oxide materials are difficult to integrate and grow with high quality. In particular metallic Heusler compounds can be deposited with industrially compatible preparation methods (sputtering), showing their technological potential for spintronics in general. However, it is not clear, whether the predicted high magnetoresistance effects were not seen because the materials are contrary to predictions not half-metals or owing to the tunnel junction properties. Especially the pronounced reduction of the magnetoresistances at room temperature is surprising, because the Curie temperatures of Heusler compounds can approach 1,000 K (for example, Co 2 MnSi [20] , [21] ). Thus there is a clear need for direct, device independent investigations of the spin polarization of Heusler compounds to clarify the intrinsic spin polarization at room temperature as this will govern the ultimate device performance. In addition, since the expectation of half-metallicity in Heusler compounds is based on band structure calculations, it is necessary to compare the theoretical with the experimental results not just concerning the single quantity of spin polarization, but concerning all electronic states of the valence band. This includes the question if Heusler materials are really half-metals. Direct experimental evidence for this property is scarce even at low temperatures for example, the highest published value obtained by point contact spectroscopy amounts to only 75% (ref. 22 ). A powerful direct spectroscopic method for the investigation of electronic band structures and spin polarizations is photoemission spectroscopy, where a photon excites an electron which is emitted and energy analyzed. The electron is excited from an initial bulk or surface state into a final state which is a free electron outside the sample and a Bloch or damped surface state inside the sample. Ultraviolet-photoemission spectroscopy (UPS) is a surface sensitive method with an information depth of ≈2 nm requiring clean and well-ordered surfaces, which, for Heusler compounds, cannot be obtained by surface cleaning procedures of ex situ prepared samples. Such attempts never resulted in relevant spin polarizations or features which could be related to the electronic band structure (for example, ref. 23 ). Also recent spin resolved UPS (SRUPS) on an ex situ prepared MgO capped Co 2 MnSi thin film measured a spin polarization of only ≃ 35% (ref. 24 ). By less surface sensitive hard X-ray photoemission spectroscopy (HAXPES, information depth ≈20 nm), the identification of intensity features with the density of states (DOS) was possible [10] , [25] , but owing to the low intensities of HAXPES no spin resolved results can be obtained. We recently demonstrated that by in situ SRUPS on epitaxial Heusler thin films the problem of surface degradation can be solved. Investigating Co 2 MnGa thin films a spin polarization of 55% at room temperature was measured in agreement with bulk band structure calculations [26] . In the following, we use this newly developed technique to investigate the compound Co 2 MnSi, which is predicted to be a half-metal. Co 2 MnSi thin film preparation and characterization Co 2 MnSi samples were prepared and investigated completely in situ in an ultrahigh vacuum cluster consisting of sputtering chambers, an molecular beam epitaxy (MBE) chamber, and a SRUPS chamber equipped with a He gas discharge lamp ( hν =21.2 eV) and a hemispherical energy analyzer with multi-channel spin filter [27] (energy resolution ≃ 400 meV, Sherman function S =0.42±0.05 (ref. 28) [28] ). First, an epitaxial buffer layer of the Heusler compound Co 2 MnGa (30 nm) was grown on the MgO(100) substrate by radio frequency (RF)-sputtering at room temperature. By an optimized additional annealing process at 550 °C L2 1 order is obtained as shown by high energy electron diffraction (RHEED) and X-ray diffraction (XRD). Co 2 MnSi (70 nm) was RF-sputtered on top at room temperature. Induced by the buffer layer the Co 2 MnSi thin films show already some degree of L2 1 surface order as deposited. By additional annealing the order is improved as demonstrated for the film surface by RHEED ( Fig. 1 ). Already a low annealing temperature of T a =300°C results in a significantly increased intensity of the characteristic RHEED L2 1 superstructure peaks. However, by XRD no (111) peak, which is indicative for L2 1 order, is observed for T a <400 °C. This suggests that L2 1 order is present at the film surface, but not in the bulk of the thin film. For T a ≥400 °C the (111) peak appears in XRD. For T a ≥500 °C some Ga from the buffer layer is observed by core-level HAXPES to have diffused to the Co 2 MnSi surface. The magnetic moments of all samples amount to ≃ 5 μ B per formula unit at 4 K and is reduced by ≃ 3% at room temperature, in agreement with theoretical predictions and experimental values measured on bulk samples [29] . 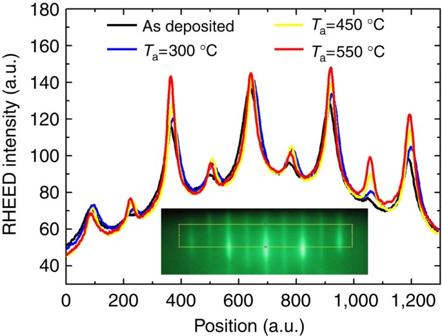Figure 1: RHEED intensities of Co2MnSi (100) thin films. The intensities for samples with different annealing temperaturesTaare evaluated from the area of the RHEED image indicated by the yellow rectangle in the inset. The inset shows the 0th order region of the RHEED image of a Co2MnSi thin film annealed at 450 °C. The low intensity maxima indicate the doubling of the unit cell (compared with the B2 cell) generated by L21order. Figure 1: RHEED intensities of Co 2 MnSi (100) thin films. The intensities for samples with different annealing temperatures T a are evaluated from the area of the RHEED image indicated by the yellow rectangle in the inset. The inset shows the 0th order region of the RHEED image of a Co 2 MnSi thin film annealed at 450 °C. The low intensity maxima indicate the doubling of the unit cell (compared with the B2 cell) generated by L2 1 order. 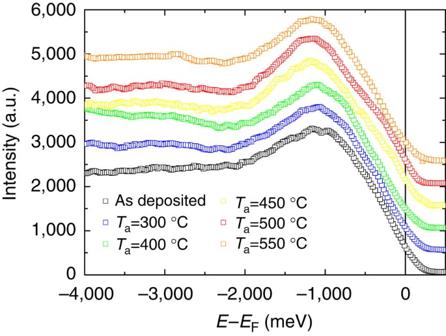Figure 2:In situspin-integrated UPS of Co2MnSi thin films. The samples were deposited at room temperature and annealed at different temperaturesTa. Curves are offset for clarity. Energy resolution ΔE=400 meV. Full size image Photoemission spectroscopy experiments Figure 2 shows in situ UPS spectra of Co 2 MnSi thin films annealed at different temperatures T a without spin analysis. The large acceptance angle of the spectrometer (±10°) and applied sample bias voltage of −10 V result in k || values which cover the complete Brillouin zone. The spectra of all samples are almost identical, only the broad hump at E − E F =−2,900 meV vanishes and the peak at E − E F =−1,150 meV is slightly broadened for the deposited and the T a =550 °C sample. Figure 2: In situ spin-integrated UPS of Co 2 MnSi thin films. The samples were deposited at room temperature and annealed at different temperatures T a . Curves are offset for clarity. Energy resolution Δ E =400 meV. Full size image However, by spin analysis clear differences between the samples are revealed. 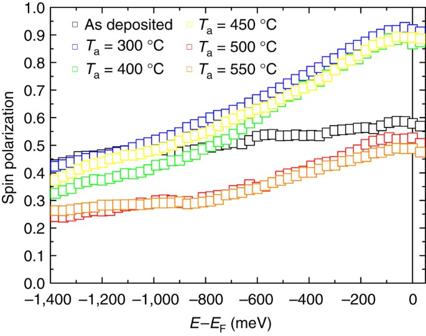Figure 3: Spin polarization determined byin situspin resolved UPS. The Co2MnSi thin films were deposited at room temperature and annealed at different temperaturesTa. The error of the Sherman functionS=0.42±0.05 (ref. 28)28results in a relative error of 12% of the spin polarization. Figure 3 shows the spin polarization of MgO/Co 2 MnGa(30 nm)/Co 2 MnSi(70 nm) thin films annealed at different temperatures T a as measured by SRUPS. A huge room temperature spin polarization of 90–93% at the Fermi energy at room temperature was obtained for samples annealed between 300 °C and 450 °C. In combination with the UPS calculations discussed below, these exceptionally high values are the first direct observation of half-metallicity in the surface region of any Heusler compound, which provide strong evidence for 100% spin polarization in the bulk of the thin films. With lower annealing temperatures the spin polarization is reduced at E F and slightly increased at higher binding energies, which can be explained by an energy broadening of the electronic states owing to reduced structural order. With higher annealing temperatures the spin polarization is reduced as a result of interdiffusion with the buffer layer. Figure 3: Spin polarization determined by in situ spin resolved UPS. The Co 2 MnSi thin films were deposited at room temperature and annealed at different temperatures T a . The error of the Sherman function S =0.42±0.05 (ref. 28) [28] results in a relative error of 12% of the spin polarization. Full size image UPS is a surface sensitive method and thus the results cannot be directly associated with electronic bulk band structure properties. However, as will be shown below, band structure based calculations of photoemission spectra provide this link. As additional experimental input for such calculations, a comparison of spin-integrated ex situ HAXPES with a photon energy of 6 keV of AlO x capped (oxidation protection) Co 2 MnSi thin films and spin-integrated in situ UPS (uncapped films) was carried out. Owing to the increased information depth of HAXPES, true surface states are typically not observed by this method. As shown in Fig. 4 , the in situ spin-integrated UPS and the HAXPES results fundamentally agree although the information depth of both experiments varies from 2 nm to 20 nm. This provides evidence that true surface states like Shockley or Tamm states, which are mainly located at the first atomic layer [30] , do not contribute to the UPS data. 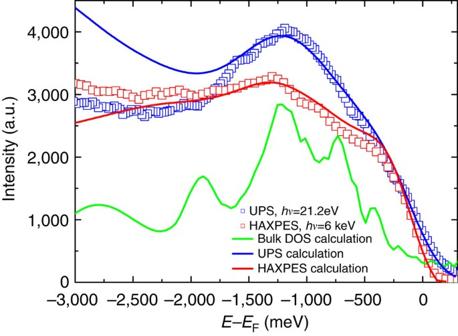Figure 4: Comparison of spin-integratedin situUPS andex situHAXPES. The Co2MnSi thin film for theex situHAXPES was capped by 2 nm AlOx(sample forin situUPS uncapped). Please note the different energy resolutions of the UPS (ΔE=400 meV) and HAXPES (ΔE=200 meV) experiments. Additionally, the spin and k-space integrated DOS as calculated using the SPR-KKR package with Perdew–Burke–Ernzerhof functional and dynamical mean field theory (UMn=3.0 eV,UCo=1.5 eV) is shown, which provides the basis for the UPS/HAXPES intensities calculated within a one-step model of photoemission (see text). The systematic deviations between calculations and measurements at higher binding energies are presumably associated with the energy-dependent detector efficiencies of the spectrometers. Figure 4: Comparison of spin-integrated in situ UPS and ex situ HAXPES. The Co 2 MnSi thin film for the ex situ HAXPES was capped by 2 nm AlO x (sample for in situ UPS uncapped). Please note the different energy resolutions of the UPS (Δ E =400 meV) and HAXPES (Δ E =200 meV) experiments. Additionally, the spin and k-space integrated DOS as calculated using the SPR-KKR package with Perdew–Burke–Ernzerhof functional and dynamical mean field theory ( U Mn =3.0 eV, U Co =1.5 eV) is shown, which provides the basis for the UPS/HAXPES intensities calculated within a one-step model of photoemission (see text). The systematic deviations between calculations and measurements at higher binding energies are presumably associated with the energy-dependent detector efficiencies of the spectrometers. Full size image Bulk DOS and photoemission calculations We calculated the spin resolved bulk DOS of Co 2 MnSi using the spin polarized relativistic Korringa–Kohn–Rostoker (SPR-KKR) Green function method implemented in the Munich SPR-KKR band structure programme package employing the Perdew–Burke–Ernzerhof functional [31] . 100% spin polarization was obtained with the gap edges at ≈−200/+200 meV. Adding correlation effects by means of dynamical mean field theory to Perdew–Burke–Ernzerhof functional [32] shifts the upper edge to higher energies, but leaves the lower edge almost unchanged. For a comparison of our experimental data with UPS- and HAXPES calculations this electronic structure provides the basis for a one-step model of photoemission, which includes all matrix-element effects, multiple scattering in the initial and final states [33] , and all surface-related effects in the excitation process. We used a recently developed relativistic generalization for excitation energies ranging from about 10 eV to more than 10 keV (ref. 34 ) realized in the full spin-density matrix formulation for the photocurrent [35] . In Fig. 4 the calculations and the experimental spin-integrated UPS and HAXPES results are compared. Nearly quantitative agreement for both, UV and hard X-ray photon energies, is obtained. Particularly with regard to the small DOS just below the Fermi energy the agreement of the calculations with the high UPS and HAXPES intensities in this energy range is remarkable and is traced back to a bulk-like surface resonance as will be discussed below. The obtained agreement between the spin-integrated UPS/HAXPES experiments and calculations based on a half metallic bulk band structure represents already evidence for half-metallicity. Additional strong evidence is provided by the analysis of the SRUPS data. For the surface region we can estimate the position of the lower band edge of the minority gap directly from the experimental data by taking the maximum of the derivative of the minority spin intensity with respect to the energy, which is found at E − E F ≃ −500 meV. From previous surface sensitive X-ray magnetic circular dichroism experiments we estimated the position of the upper band edge to be at E − E F ≃ +400 meV (ref. 36 ). In Fig. 5 the highest experimentally obtained spin polarization is shown together with the spin polarization derived directly from the calculated DOS, the calculated photoemission asymmetry including all broadening effects considering bulk contributions only, and the calculated photoemission asymmetry including surface-related effects. The correspondence between the DOS and calculated pure bulk-like UPS spectrum becomes clear, if the influence of intrinsic life time broadening owing to electronic correlations and included experimental energy resolution (Δ E =400 meV) is considered. It is obvious that these broadening effects within the bulk calculations reduce the expected UPS spin polarization although the DOS is half-metallic. However, including surface effects in the calculation changes the results clearly. 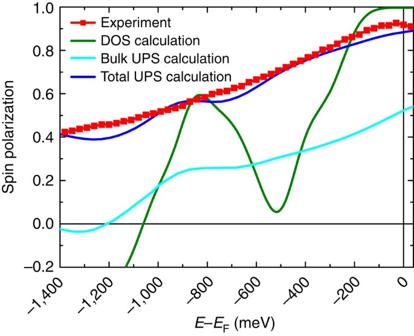Figure 5: Calculated and experimental spin polarizations. Comparison of the spin polarization obtained byin situSRUPS on a Co2MnSi thin film with the calculated DOS-derived spin polarization, the calculated UPS spin polarization including broadening effects and considering only bulk states, and the calculated total UPS spin polarization including broadening effects with additional surface state contributions. The theoretical curves were obtained using the SPR-KKR package with Perdew–Burke–Ernzerhof functional and dynamical mean field theory. The error of the Sherman functionS=0.42±0.05 (ref. 28)28results in a relative error of 12% of the spin polarization. Figure 5: Calculated and experimental spin polarizations. Comparison of the spin polarization obtained by in situ SRUPS on a Co 2 MnSi thin film with the calculated DOS-derived spin polarization, the calculated UPS spin polarization including broadening effects and considering only bulk states, and the calculated total UPS spin polarization including broadening effects with additional surface state contributions. The theoretical curves were obtained using the SPR-KKR package with Perdew–Burke–Ernzerhof functional and dynamical mean field theory. The error of the Sherman function S =0.42±0.05 (ref. 28) [28] results in a relative error of 12% of the spin polarization. Full size image True surface states contribute to the layer-resolved photocurrent with an intensity distribution that is nonzero for the first atomic layer only. Consequently, their contribution to the total spectral weight decreases with increasing number of layers generating the photocurrent. Thus in general with increasing photon energies the combined effect of energy-dependent cross-sections and larger inelastic mean free path results in a reduced weight of surface state photoemission. However, the situation is very different for Co 2 MnSi, where we identified in our calculations a resonance on the (001)-surface, which is embedded in the bulk continuum with a strong coupling to the majority bulk states. In our case this surface resonance extends over the first six atomic layers, which is similar to the case of W(110), where we found a surface resonance revealing a considerable bulk contribution [35] as well. The spectral weight of this surface resonance is much larger than that of a true surface state resulting in a significant contribution to the total intensity even at hard X-ray energies. As shown in Fig. 5 , the inclusion of the complete surface-related photoexcitation in the UPS calculation results in perfect agreement with the experiment. If the surface resonance were not present, half-metallic behaviour would persist but the finite experimental resolution in photoemission would hinder the observation of a high spin polarization. Because the surface resonance is strongly coupled to the band structure of the bulk, this provides evidence for the validity of our calculated half metallic bulk band structure of Co 2 MnSi. And, from the spintronics applications point of view it is the room temperature spin polarization in the thin film surface region, which is relevant. In conclusion, investigating optimized thin films of the compound Co 2 MnSi by in situ SRUPS, we were able to demonstrate for the first time half-metallicity in combination with directly measured ( ) % spin polarization at room temperature in the surface region of a Heusler thin film. Novel band structure and photoemission calculations including all surface-related effects show that the observation of a high spin polarization in a wide energy range below the Fermi energy is related to a stable surface resonance in the majority band of Co 2 MnSi extending deep into the bulk of the material. Our results show that careful thin film preparation can indeed result in a high spin polarization with a sufficient degree of stability in a surface region of several atomic layers. In particular it shows that the observed tunnelling magnetoresistance values are not limited by the intrinsic spin polarization of the Heusler alloy and that potentially much larger values can be obtained by carefully optimized growth. Fundamentally our observation paves the way for most powerful future spintronic devices on the basis of Heusler materials. How to cite this article: Jourdan, M. et al. Direct observation of half-metallicity in the Heusler compound Co 2 MnSi. Nat. Commun. 5:3974 doi: 10.1038/ncomms4974 (2014).